Alkyl halides as both hydride and alkyl sources in catalytic regioselective reductive olefin hydroalkylation Among the plethora of catalytic methods developed for hydrocarbofunctionalization of olefins to date, reactions that regioselectively install a functionalized alkyl unit at the 2-position of a terminal unactivated C=C bond to afford branched products are scarce. Here, we show that a Ni-based catalyst in conjunction with a stoichiometric reducing agent promote Markovnikov-selective hydroalkylation of unactivated alkenes tethered to a recyclable 8-aminoquinaldine directing auxiliary. These mild reductive processes employ readily available primary and secondary haloalkanes as both the hydride and alkyl donor. Reactions of alkenyl amides with ≥ five-carbon chain length regioselectively afforded β-alkylated products through remote hydroalkylation, underscoring the fidelity of the catalytic process and the directing group’s capability in stabilizing five-membered nickelacycle intermediates. The operationally simple protocol exhibits exceptional functional group tolerance and is amenable to the synthesis of bioactive molecules as well as regioconvergent transformations. The abundance, low cost and distinct reactivity profiles of alkenes have enabled these feedstock molecules to be widely utilized in olefin functionalization reactions for various chemical synthesis applications [1] , [2] , [3] . In this respect, the installation of a hydrogen and carbon-based moiety across π-systems represents an effective strategy for C–C bond construction [4] , [5] , [6] . Numerous hydrocarbofunctionalization protocols rely on conjugation (i.e., 1,3-dienes [7] , [8] , [9] , [10] , [11] , olefins such as styrenes [12] , [13] , [14] , alkenyl boronates [15] , [16] , and Michael acceptors [17] ) to deliver high regioselectivity. In contrast, reactions with unactivated aliphatic C=C bonds are typically plagued by lower substrate reactivity and/or poorer regiochemical differentiation leading to unsatisfactory levels of site selectivity. Notwithstanding these difficulties, remarkable advances for both anti-Markovnikov [18] , [19] , [20] , [21] , [22] , [23] , [24] , [25] (linear)- and Markovnikov [26] , [27] , [28] , [29] , [30] (branched)-selective hydroarylations of alkyl-substituted alkenes have been made. A single report on Pd-catalyzed olefin hydroalkynylation/hydroalkenylation to afford linear products was also recently disclosed [31] . On the other hand, there is growing demand for methods that furnish C–C bonds between two sp 3 -hybridized motifs, which are crucial for assembling the skeletal backbone of organic entities en route to bioactive compounds [32] , [33] . Accordingly, hydroalkylations across aliphatic olefins have been devised, although the vast majority involved linear-selective additions (Fig. 1a ). Of these cases, either a limited range of ureas [34] , organometallic reagents [35] , [36] or carbonyl compounds [37] , [38] , [39] were employed as nucleophiles, or an exogenous protic source [40] or hydrosilane/base reagent [41] , [42] , [43] , [44] , [45] is needed to (i) promote protodemetallation or (ii) generate the requisite metal-hydride species. Fig. 1: The significance of developing branched- and β-selective hydroalkylation of unactivated alkenes. a Reported methods that involve anti-Markovnikov-selective hydroalkylation of aliphatic olefins. b Reported methods that involve Markovnikov-selective hydroalkylation of aliphatic olefins. c An attractive catalytic approach for Markovnikov- and β-selective olefin hydroalkylation takes advantage of haloalkanes to transfer the hydride and alkyl motif under mild reductive conditions without additional hydrosilane, acidic or basic additives. d The resulting hydroalkylation products are versatile building blocks that may be used to access biologically active molecules. R, functional group; Phth, phthaloyl; pyr., pyridinium; cat., catalyst. Full size image To date, highly Markovnikov-selective hydroalkylations of aliphatic π-systems have been largely achieved with 1,1-disubstituted/trisubstituted alkenes and primary haloalkanes through a Mn/Ni dual catalytic metal-hydride hydrogen atom transfer approach [46] , or with olefins linked to a tridendate directing group and 1,3-dicarbonyl nucleophiles using a Pd-based catalyst [40] (Fig. 1b ). Therefore, there is compelling motivation to develop a complementary catalytic regime that accomplishes efficient and branched-selective hydroalkylation of unactivated acyclic olefins with exceptional control of regioselectivity in the presence of commonly occurring functionalities. For operational simplicity, we speculated that aliphatic halides could serve as mild donors of both the hydride (by facile in situ β-H elimination [47] , [48] ) and alkyl component without external acidic or basic additives, which might otherwise compromise functional group compatibility (Fig. 1c ). The products resulting from successful implementation of this strategy can be readily elaborated to a variety of important biologically active compounds (e.g., 1 – 3 , Fig. 1d ). Herein, we report a directed Ni-catalyzed reductive protocol that achieves these goals. Reaction design and optimization A hallmark of catalytic reductive transformations [49] , [50] , [51] , [52] , [53] , [54] , [55] , [56] , [57] is the use of stoichiometric amounts of an inexpensive reducing agent to drive single-electron transfer processes mediated by an appropriate (e.g., Ni-based) catalyst. This led us to conceive a reductive strategy for alkene hydroalkylation that takes advantage of the characteristic mild reaction conditions. Specifically, we aimed to avoid the use of hydrosilanes, acidic and basic reagents that could engender undesired side reactions with certain sensitive functional units (see below for further discussion). However, the question remains how we could effectively deliver hydride to the C=C bond in this scenario. To this end, we envisioned a catalytic approach that merges aliphatic alkenes tethered to a suitable directing unit 4 [58] with alkyl halides directly in the presence of a Ni-based catalyst and a reductant (Fig. 2 ). This strategy relies on the propensity of haloalkanes to undergo facile β-H elimination, an observation that was previously exploited in Ni catalysis to generate catalytic amounts of nickel-hydride species [47] , [48] . As illustrated in the putative catalytic pathway, a Ni(0) species i could first associate with 4 and react with an equivalent of the alkyl halide through a halogen atom abstraction/radical recombination [59] , [60] process to give ii . At this juncture, a directing auxiliary with appropriate steric and/or electronic properties could induce alkene dissociation from the metal center in ii , providing an opportunity for the Ni–alkyl moiety to preferentially undergo β-H elimination [47] , [48] leading to nickel-hydride iii with concomitant discharge of an alkene by-product (vs. olefin alkylnickelation to form viii ). Regioselective β-hydride insertion across the associated C=C bond in iii then affords quinoline-chelated Ni(II) species iv . Following single-electron reduction with a reducing agent, Ni(I) complex v would be generated that could subsequently react with a second equivalent of alkyl halide to furnish vi . Reductive elimination of vi furnishes the desired hydroalkylation product 5 and vii , which eventually gets reduced back to i to turn over the catalytic cycle. The key to efficient transformation of 4 to 5 entails faster conversion of intermediate ii to iv via iii (vs. ii to viii ) in order to suppress adventitious formation of the undesired dialkylation adduct 6 . Fig. 2: The challenges involved in developing site-selective reductive hydroalkylation reactions. As shown in the Ni catalytic cycle, the key to efficient transformation of 4 to 5 requires faster conversion of intermediate ii to iv in order to suppress adventitious formation of the undesired dialkylation adduct 6 . Under the reductive conditions, both the hydrogen and alkyl unit are derived from the haloalkane reagent. R, G, functional group; X, halide; L, ligand; cat., catalyst. 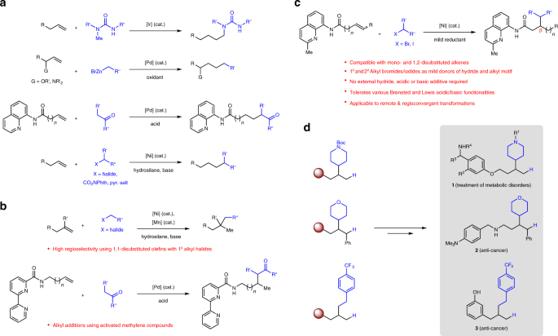Fig. 1: The significance of developing branched- and β-selective hydroalkylation of unactivated alkenes. aReported methods that involve anti-Markovnikov-selective hydroalkylation of aliphatic olefins.bReported methods that involve Markovnikov-selective hydroalkylation of aliphatic olefins.cAn attractive catalytic approach for Markovnikov- and β-selective olefin hydroalkylation takes advantage of haloalkanes to transfer the hydride and alkyl motif under mild reductive conditions without additional hydrosilane, acidic or basic additives.dThe resulting hydroalkylation products are versatile building blocks that may be used to access biologically active molecules. R, functional group; Phth, phthaloyl; pyr., pyridinium; cat., catalyst. Full size image We first examined conditions that facilitate hydroalkylation of β,γ-unsaturated amides with 1-iodobutane 8 (Table 1 ). After an extensive survey, we found that the reaction between 8-aminoquinaldine-tethered alkene 7a and 8 (2 equiv.) using NiCl 2 (PPh 3 ) 2 (15 mol%), manganese (1.5 equiv.) as reductant and NMP as solvent gave the best results, affording 9a in 90% GC (88% isolated) yield and complete Markovnikov selectivity at ambient temperature (Table 1 , entry 1). There was no appreciable diminution in yield or selectivity when the reaction was carried out on larger scale (2 mmol). Intriguingly, changing the directing group to other variants gave poorer yields and site selectivities, demonstrating the unexpected beneficial role of the ortho -methyl appendage. We reasoned that the effect might arise from an elevated steric strain inherent within complex ii (cf. Fig. 2 ), forcing Ni-olefin dissociation and allowing the sterically less demanding C β –H bond to coordinate and trigger β-H elimination [47] , [48] prior to the ensuing β-H insertion to iv . Further studies to rationalize this effect will be reported in due course. Table 1 Evaluation of reaction conditions for reductive hydroalkylation. Full size table Changing the Ni-based catalyst afforded lower yields across the board (Table 1 entry 2), while replacing NMP with other solvents did not improve results (Table 1 , entries 3–4). Unsurprisingly, the reaction did not proceed in the absence of Mn, with 1.5 equiv. of Mn being optimal (Table 1 , entries 5–7). Switching Mn to Zn as the reductant led to a drastic reduction in yield and regioselectivity (Table 1 entry 8). Decreasing the equivalents of 8 resulted in diminished reaction efficiency, whereas no appreciable improvement was detected at higher loadings (Table 1 entries 9–10). Carrying out the reaction at 40 °C gave similar results as RT (Table 1 , entry 11). A slight drop in site selectivity was observed with 10 mol% loading of NiCl 2 (PPh 3 ) 2 (Table 1 , entry 12). Performing the hydroalkylation by replacing Mn with hydrosilane/base as the hydride source [41] , [42] , [43] , [44] , [45] led to lower yields of 9a (see Supplementary Methods 2.6 for details), highlighting the importance of the reductive conditions. Substrate scope With the established conditions in hand, we proceeded to evaluate the scope by examining various functionalized aliphatic halides and alkenyl amides (Fig. 3 ). Primary alkyl iodides and bromides containing different functional groups underwent efficient hydroalkyl additions to 7a , furnishing the desired branched compounds 9b – w in 32–94% yield and high regioselectivities. Transformations with less activated organobromides were performed at 60 °C for optimal efficiency. These include products that contain an ester ( 9d ), an enoate ( 9e ), an aldehyde ( 9h ), an alkene ( 9n ) as well as unprotected protic units (problematic with basic organometallic reagents) [57] , [61] such as carboxylic acid ( 9k ), alcohol ( 9p – q ) and phenol ( 9r ). It merits mention that previous methods which rely on hydrosilane/base to generate the hydride source may cause undesired silylation side reactions with hydroxyl groups [46] . Both acid-labile (acetal 9o ) and base-labile ( 9k , 9r and boronate 9t ) functionalities, which could be vulnerable under conditions that require acid/base additives [40] , [41] , [42] , [43] , [44] , [45] , [46] , as well as Lewis basic heterocyclic motifs ( 9f , 9u – v ) are tolerated. Among the products bearing a derivatizable halogen appendage ( 9i – j , 9s ), the reaction that afforded 9j highlights the inherent chemoselectivity of an iodoalkane over an aryl iodide, although arene hydrodeiodination was detected as a side reaction. The reductive protocol is also compatible with substrates derived from complex multifunctional bioactive molecules such as base-sensitive sulbactam [62] ( 9l ) and indometacin ( 9m ). Fig. 3: The range of products accessible by reductive olefin hydroalkylation. The protocol is compatible with both primary and secondary alkyl halides bearing Brønsted/Lewis acidic and basic functionalities, including those derived from complex bioactive molecules. Both mono- and 1,2-disubstituted alkenyl amides are tolerated in the catalytic system. For 9w , the reaction was conducted with neopentyl bromide (3 equiv.) and isopropyl bromide (1.2 equiv.) using NiI 2 as the catalyst. For 9ac and 9af , reactions were conducted using iodides (X = I). For 9ad , 9ae , and 9ag , reactions were conducted using bromides (X = Br). For 9j , ~20% of an inseparable hydrodeiodination side product was detected. For 9m , ~3% of an inseparable self-coupling side product of iodide substrate was detected. 9g , 9i , 9u , 9ab , and 9af were obtained as 88:12, 93:7, 92:8, 90:10, and 91:9 regioisomeric mixtures, respectively. 9l and 9z were obtained as 5:1 and 1:1 diastereomeric mixtures, respectively. Regioisomeric and diastereomeric ratios were determined by 1 H NMR analysis. Yields are for isolated and purified products. R, functional group; X, halide; NMP, N -methyl-2-pyrrolidone; Boc, tert -butoxycarbonyl. Full size image Secondary alkyl iodides and bromides also served as effective reagents under the standard conditions, delivering the expected products 9x – ab in 51–73% yield and offering complementary scope to a previous report in which secondary haloalkanes were low-yielding [46] . However, organohalides that lack a C β –H bond and therefore incapable of generating the requisite nickel-hydride species by β-H elimination pose a challenge in our system. Attempts to carry out reductive hydroalkylation using neopentyl bromide (3 equiv.) as alkyl donor and isopropyl bromide (1.2 equiv.) as hydride donor [47] , [48] gave the desired hydroalkylation adduct 9w in 32% yield, along with side products derived from dialkylation with neopentyl bromide as well as reductive hydroalkylation with isopropyl bromide (see Supplementary Methods 2.7 for details). β,γ-Unsaturated amides with 1,2-disubstitiuted C=C bonds underwent reaction to form the corresponding β-alkylated products ( 9ac – ag ), but those with 1,1-disubstituted and trisubstituted olefins were ineffective substrates (<5% conv. to desired product). Synthetic applications The first application that demonstrates utility of our Markovnikov-selective reductive hydroalkylation protocol involves the synthesis of a family of therapeutic compounds 1 for the treatment of metabolic disorders [63] (Fig. 4a ). Chemoselective removal of the amide directing group in 9y (recovered 8-aminoquinaldine in 95% yield) afforded acid 11 , a key intermediate employed in the preparation of 1 , in 83% yield. Fig. 4: Application to synthesis of biologically active molecules and remote hydroalkylation. a The products resulting from reductive hydroalkylation can be conveniently transformed to a variety of medicinal compounds of interest. b Alkenyl amides bearing ≥ five-carbon chain length undergo remote hydroalkylation through in situ isomerization of alkylnickel intermediates, providing reliable access to β-alkylated molecules. Regioisomeric olefin mixtures can be regioconvergently converted to a single value-added product. Regioisomeric ratios were determined by 1 H NMR analysis. Yields are for isolated and purified products. 9ah was obtained as a 96:4 regioisomeric mixture. For 18a , 18d , 18e , and 18g , reactions were conducted using iodides (X = I). For 18b , 18c , and 18f , reactions were conducted using bromides (X = Br). For 18g , 5 equiv. of 1-iodobutane was used. R, functional group; X, halide; NMP, N -methyl-2-pyrrolidone; DMA, N , N -dimethylacetamide; NHPI, N -hydroxyphthalimide; DIC, N , N ′-diisopropylcarbodiimide; DMAP, 4-dimethylaminopyridine; dtbbpy, 4,4′-di- tert -butyl-2,2′-bipyridine; Boc, tert -butoxycarbonyl; Phth, phthaloyl; Cp, cyclopentadienyl; RT, room temperature. Full size image In a second instance, chemoselective reduction of the 8-aminoquinaldine amide in 9ah to aldehyde 12 followed by reductive amination with benzylamine 13 and N -Boc protection delivered 14 , a precursor for the synthesis of an anti-cancer compound 2 [64] , in 51% overall yield. The entire sequence is more concise compared to a previous report [64] . The preparation of 16 highlights yet another compelling example of the versatility of the branched hydroalkylation products. Facile conversion of 9ai to its redox-active ester derivative 15 (70% overall yield) set the stage for a catalytic decarboxylative cross-coupling [53] with 1-(benzyloxy)-3-iodobenzene to furnish 16 , which has been further elaborated to another anti-cancer agent 3 [65] . A corollary to the present reductive approach is the implementation of remote olefin hydroalkylation [66] , [67] , [68] , [69] , [70] , specifically with alkenyl amides 17 containing an extended hydrocarbon backbone (≥ five-carbon chain length). As showcased in Fig. 4b , we postulated that the organonickel intermediate ix generated from nickel-hydride addition (cf. Fig. 2 ) could potentially isomerize to the relatively more stabilized five-membered nickelacycle x [66] , [67] , [71] through consecutive β-H elimination/olefin insertion steps. Following a similar mechanism in Fig. 2 , x could be converted to 18 with net remote alkylation at the β position. Although nickel-hydride-promoted remote hydrocarbonfunctionalizations have been disclosed, most instances involve functionalizations at either the sterically exposed terminus or the α-carbon site adjacent to an electron-stabilizing moiety [68] , [69] . Gratifyingly, γ,δ-unsaturated amides bearing terminal and internal C=C bonds were found to participate in remote hydroalkylation with primary and secondary haloalkanes, affording products 18a – e in 47–82% yield as single β regioisomers through single double-bond migrations (Fig. 4b ). Cyclic olefins also underwent reaction as exemplified by 18e , which was obtained as a single syn diastereomer [71] . Using the regioisomeric β,γ-unsaturated amide substrate leading to 18e would be, however, less practical since the corresponding β,γ-unsaturated carboxylic acid is much more expensive. Transformations with δ,ε-unsaturated amides (involving two C=C bond isomerizations) were similarly efficient and site-selective ( 18d and 18f ). Remarkably, subjecting the 6-heptenoic acid-derived alkenyl amide to established conditions gave β-alkylated 18g in 60% yield, underscoring the fidelity of the catalytic process that features an alkene transposition over three positions [67] , [68] . Furthermore, a streamlined synthesis of β-alkylated 18d could be attained in 62% yield through regioconvergent hydroalkylation of an isomeric mixture of olefin substrates (Fig. 4b , gray inset). Mechanistic studies Subjecting the α,β-unsaturated isomer of 7a to the standard conditions only gave the fully hydrogenated product 19 , thereby ruling out the likelihood of olefin isomerization prior to the hydroalkylation event (Fig. 5a ). To shed light on the importance of the alkyl halide partner in our catalytic system, we carried out deuterium labeling studies with 7a in the presence of two equivalents of d - 20 under the standard reaction conditions (Fig. 5b ). Accordingly, the hydroalkylation product d - 9aj and olefin by-product d - 21 were isolated. Deuterium incorporation on C1 of d - 9aj and deuterium scrambling in d - 21 suggest that a nickel-deuteride species was likely generated from reaction with d - 20 (i.e., ii → iii in Fig. 2 ). The reversible nature of β-H(D) elimination and re-insertion means that adventitious deuterium scrambling in d - 21 and formation of Ni–H cannot be avoided. Competitive addition of Ni–H and Ni–D across the olefin in 7a eventually gave rise to d - 9aj with 40% D incorporation at C1. Overall, these results support the haloalkane’s key role as a donor of both the hydride and alkyl group. Fig. 5: Mechanistic studies. a Control experiment ruling out the intermediacy of 7a′ . b Deuterium labeling experiment. c Radical clock experiment. d Complete stereochemical erosion with an enantioenriched alkyl halide. Diastereomeric ratios were determined by 1 H NMR analysis. Enantiomeric ratios were determined by chiral HPLC analysis. Yields are for isolated and purified products. NMP, N -methyl-2-pyrrolidone; RT, room temperature. Full size image The radical nature of the reductive hydroalkylation reaction was substantiated through a radical clock experiment using (bromomethyl)cyclopropane 22 as an electrophile (Fig. 5c ). A 20:80 mixture of 9ak and the ring-ruptured product 9n in 84% yield was detected, intimating that 22 likely reacts with the catalytic organonickel species (cf. i → ii and v → vi in Fig. 2 ) through a bromine abstraction/radical recombination process [59] , [60] via a cyclopropylmethyl radical that is prone to ring opening. Further support for the intermediacy of radicals could be obtained from the corresponding reactions using enantioenriched 23 , in which the desired product 9al was generated in 51–73% yield and ~70:30 d.r. as a racemic mixture (Fig. 5d ). In summary, we demonstrated that Ni-catalyzed branched-selective hydroalkyl additions to unactivated alkenyl amides can be achieved by using haloalkanes and manganese as reductant. With long-chain olefins, remote and regioconvergent hydroalkylations proceed to furnish products with reliable β selectivities. Mechanistic experiments corroborate the aliphatic halide’s dual role as a hydride and alkyl donor. Equally crucial is the 8-aminoquinaldine tether that effectively suppresses any adventitious dialkylation side reaction. 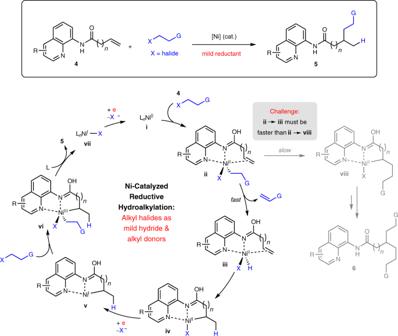Fig. 2: The challenges involved in developing site-selective reductive hydroalkylation reactions. As shown in the Ni catalytic cycle, the key to efficient transformation of4to5requires faster conversion of intermediateiitoivin order to suppress adventitious formation of the undesired dialkylation adduct6. Under the reductive conditions, both the hydrogen and alkyl unit are derived from the haloalkane reagent. R, G, functional group; X, halide; L, ligand; cat., catalyst. The robust conditions are compatible with diverse functional groups, including those that are sensitive to hydrosilane, acidic or basic additives. In conjunction with existing methods, we expect our catalytic strategy to find significant utility in chemical synthesis. 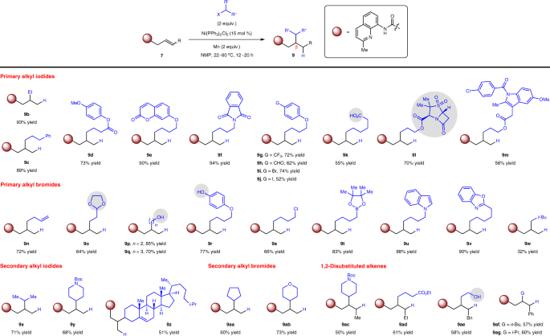Fig. 3: The range of products accessible by reductive olefin hydroalkylation. The protocol is compatible with both primary and secondary alkyl halides bearing Brønsted/Lewis acidic and basic functionalities, including those derived from complex bioactive molecules. Both mono- and 1,2-disubstituted alkenyl amides are tolerated in the catalytic system. For9w, the reaction was conducted with neopentyl bromide (3 equiv.) and isopropyl bromide (1.2 equiv.) using NiI2as the catalyst. For9acand9af, reactions were conducted using iodides (X = I). For9ad,9ae, and9ag, reactions were conducted using bromides (X = Br). For9j, ~20% of an inseparable hydrodeiodination side product was detected. For9m, ~3% of an inseparable self-coupling side product of iodide substrate was detected.9g,9i,9u,9ab, and9afwere obtained as 88:12, 93:7, 92:8, 90:10, and 91:9 regioisomeric mixtures, respectively.9land9zwere obtained as 5:1 and 1:1 diastereomeric mixtures, respectively. Regioisomeric and diastereomeric ratios were determined by1H NMR analysis. Yields are for isolated and purified products. R, functional group; X, halide; NMP,N-methyl-2-pyrrolidone; Boc,tert-butoxycarbonyl. General reductive hydroalkylation procedure In a N 2 -filled glovebox, to an oven-dried 5 mL vial equipped with a magnetic stir bar were added alkene substrate (0.1 mmol), alkyl iodide or bromide (if solid, added at this time) (0.2 mmol), Ni(PPh 3 ) 2 Cl 2 (9.8 mg, 0.015 mmol) and Mn powder (0.15 mmol). The mixture was then dissolved in 0.3 mL dry NMP. 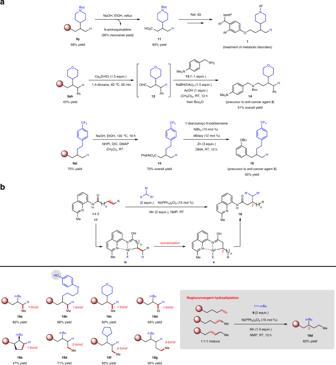Fig. 4: Application to synthesis of biologically active molecules and remote hydroalkylation. aThe products resulting from reductive hydroalkylation can be conveniently transformed to a variety of medicinal compounds of interest.bAlkenyl amides bearing ≥ five-carbon chain length undergo remote hydroalkylation through in situ isomerization of alkylnickel intermediates, providing reliable access to β-alkylated molecules. Regioisomeric olefin mixtures can be regioconvergently converted to a single value-added product. Regioisomeric ratios were determined by1H NMR analysis. Yields are for isolated and purified products.9ahwas obtained as a 96:4 regioisomeric mixture. For18a,18d,18e, and18g, reactions were conducted using iodides (X = I). For18b,18c, and18f, reactions were conducted using bromides (X = Br). For18g, 5 equiv. of 1-iodobutane was used. R, functional group; X, halide; NMP,N-methyl-2-pyrrolidone; DMA,N,N-dimethylacetamide; NHPI,N-hydroxyphthalimide; DIC,N,N′-diisopropylcarbodiimide; DMAP, 4-dimethylaminopyridine; dtbbpy, 4,4′-di-tert-butyl-2,2′-bipyridine; Boc,tert-butoxycarbonyl; Phth, phthaloyl; Cp, cyclopentadienyl; RT, room temperature. 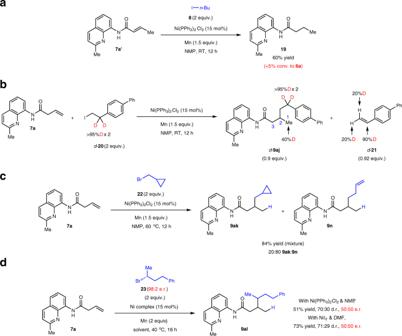Fig. 5: Mechanistic studies. aControl experiment ruling out the intermediacy of7a′.bDeuterium labeling experiment.cRadical clock experiment.dComplete stereochemical erosion with an enantioenriched alkyl halide. Diastereomeric ratios were determined by1H NMR analysis. Enantiomeric ratios were determined by chiral HPLC analysis. Yields are for isolated and purified products. NMP,N-methyl-2-pyrrolidone; RT, room temperature. The vial was tightly capped and removed from the glovebox. The alkyl iodide or bromide (if liquid, added at this time) was added by a micro-syringe. The mixture was allowed to vigorously stir at ambient temperature (for alkyl iodide) or 60 °C (for alkyl bromide) for 12–20 h. When alkene was almost fully consumed (monitored by TLC), the mixture was directly subjected to flash silica gel column chromatography to afford the pure product.